Room-temperature electronically-controlled ferromagnetism at the LaAlO3/SrTiO3interface Reports of emergent conductivity, superconductivity and magnetism have helped to fuel intense interest in the rich physics and technological potential of complex-oxide interfaces. Here we employ magnetic force microscopy to search for room-temperature magnetism in the well-studied LaAlO 3 /SrTiO 3 system. Using electrical top gating to control the electron density at the oxide interface, we directly observe the emergence of an in-plane ferromagnetic phase as electrons are depleted from the interface. Itinerant electrons that are reintroduced into the interface align antiferromagnetically with the magnetization at first screening and then destabilizing it as the conductive regime is approached. Repeated cycling of the gate voltage results in new, uncorrelated magnetic patterns. This newfound control over emergent magnetism at the interface between two non-magnetic oxides portends a number of important technological applications. Vigorous efforts have been made to integrate magnetism with semiconductors [1] , [2] , [3] . Ideally, a ferromagnetic semiconductor would possess full electrical control over its magnetic properties combined with strong coupling to the spin of mobile charge carriers. Efforts to identify suitable materials have focused on diluted magnetic semiconductors such as (Ga,Mn)As [4] , diluted magnetic oxides [3] and magneto-electric materials such as chromia [5] . Strong electronic correlations [6] can also induce charge-ordered phases, produce electronic phase separation and stabilize various types of magnetic order. The two-dimensional electron liquid (2DEL) that forms at the interface between the two insulating non-magnetic oxides LaAlO 3 (LAO) and SrTiO 3 (STO) [7] has drawn widespread attention due to its possession of a remarkable variety of emergent behaviour including superconductivity [8] , strong Rashba-like spin-orbit coupling [9] , [10] and ferromagnetism [11] , [12] , [13] , [14] , [15] . The first signatures of magnetism at the LAO/STO interface were reported in magneto-transport measurements by Brinkman et al . [11] Direct current scanning quantum interference device (SQUID) magnetometry measurements by Ariando et al . [12] showed ferromagnetic hysteresis extending to room temperature. Torque magnetometry measurements by Li et al . [13] showed evidence for in-plane magnetism with a high moment density (~0.3 μ B per unit cell). Scanning SQUID microscopy by Bert et al . [14] revealed inhomogeneous micron-scale magnetic ‘patches’. X-ray circular dichroism measurements by Lee et al . [15] indicate that the ferromagnetism is intrinsic and linked to d xy orbitals in the Ti t 2g band. Despite this variety of evidence, the existence and nature of magnetism in LAO/STO heterostructures has remained controversial. Neutron reflectometry measurements by Fitzsimmons et al . [16] on LAO/STO superlattices found no magnetic signatures; their measurements established a bulk upper limit thirty times lower than what was reported by Li et al . [13] Salman et al . [17] reported relatively small moments from LAO/STO superlattices (~2 × 10 −3 μ B per unit cell) using β-detected nuclear magnetic resonance. Our search for magnetism at the LAO/STO interface is guided by the fact that most of the interesting behaviour observed at the LAO/STO interface—superconductivity, spin-orbit coupling, anisotropic magnetoresistance and anomalous Hall behaviour—depends strongly on carrier density [18] , [19] , [20] , [21] . The electron density at the interface can be controlled using a number of techniques including back-gating [22] , top-gating [23] , polar adsorbates [24] or via nanoscale control using conductive atomic force microscopy (AFM) lithography [25] . In this article we investigate magnetism at the LAO/STO interface using magnetic force microscopy (MFM) [26] . By using top-gated LAO/STO heterostructures we are able to search for magnetism as a function of mobile interfacial carrier density. We directly observe the emergence of an in-plane ferromagnetic phase as electrons are depleted from the interface. Reintroducing the itinerant electrons, which align antiferromagnetically with the magnetization, into the interface at first screens and then destabilizes the magnetization as the conductive regime is approached. Experiment set-up and investigated device In this report, all measurements are performed in ambient conditions at room temperature. The sample is kept within a darkened chamber during experiments to minimize photoexcitation of carriers. LAO/STO heterostructures are fabricated by depositing 12 unit cell LAO films on TiO 2 -terminated (001) STO substrates using pulsed laser deposition with in situ high-pressure reflection high energy electron diffraction. LAO/STO heterostructures are patterned with top circular electrodes and concentric arc-shaped interfacial contacts, sketched in Fig. 1a . Details of the growth technique and device fabrication are described more fully in the Methods section. 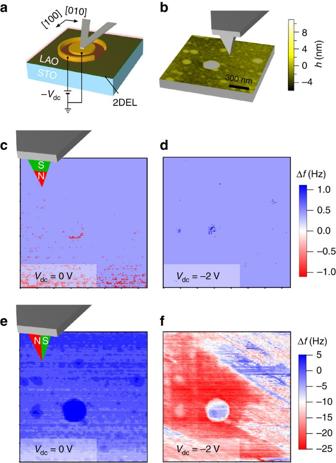Figure 1: MFM experiments on gated LaAlO3/SrTiO3heterostructures. (a) Sketch of experimental set-up. The MFM tip is mechanically driven by a piezoelectric transducer near its resonant frequency and kept at a constant heightΔhabove the surface. The top electrode and MFM tip are both grounded and a DC bias is directly applied to the interface. Frequency modulation is used to lock the phase of the mechanical response at 90°. The frequency shift Δfis proportional to the force gradient. (b) Surface topography over the investigated 1.4 × 1.4 μm area on the top electrode. (c,d) MFM frequency-shift images using vertically magnetized tip withVdc=0 and −2 V. (e,f) MFM frequency images over the same area using a tip that is magnetized horizontally along the [010] direction. Images are taken underVdc=0 and −2 V. Experimental measurements are presented for three devices whose parameters are summarized in Supplementary Table 1 . For consistency, the main results are presented for Device A. A summary of all investigated locations including the other two devices are shown in Supplementary Fig. 1 . Figure 1: MFM experiments on gated LaAlO 3 /SrTiO 3 heterostructures. ( a ) Sketch of experimental set-up. The MFM tip is mechanically driven by a piezoelectric transducer near its resonant frequency and kept at a constant height Δh above the surface. The top electrode and MFM tip are both grounded and a DC bias is directly applied to the interface. Frequency modulation is used to lock the phase of the mechanical response at 90°. The frequency shift Δ f is proportional to the force gradient. ( b ) Surface topography over the investigated 1.4 × 1.4 μm area on the top electrode. ( c , d ) MFM frequency-shift images using vertically magnetized tip with V dc =0 and −2 V. ( e , f ) MFM frequency images over the same area using a tip that is magnetized horizontally along the [010] direction. Images are taken under V dc =0 and −2 V. Full size image A two-terminal capacitor device is used to electrically gate the LAO/STO interface ( Fig. 1a ). The top circular electrode is grounded and a voltage − V dc is applied to the annular interface contact. (This configuration is equivalent to grounding the interface and applying + V dc to the top electrode). Decreasing V dc depletes the interface of mobile electrons, while increasing V dc leads to electron accumulation and results in a conductive interface. The critical voltage for the metal-insulator transition is device dependent and generally exhibits voltage hysteresis in the range −2 V to −0 V. The transition is readily identified as an inflection point in the capacitance–voltage (CV) spectrum ( Supplementary Fig. 2 ). The leakage current is device dependent ( Supplementary Fig. 3 ) and does not scale with the top electrode area, suggesting the existence of pinholes. These leakage currents are approximately eight orders of magnitude lower than what is required to generate a measurable magnetic signal [27] , [28] . A CoCr-coated AFM tip is first characterized ( Supplementary Fig. 4 ) and then magnetized ( Supplementary Fig. 5 ) with magnetic field up to 2000 Oe. A reference sample is used to verify the tip is properly magnetized ( Supplementary Fig. 6 , Supplementary Note 1 ). The AFM scanning environment is shown in Supplementary Fig. 7 . In the MFM mode, the cantilever is mechanically driven by a piezoelectric transducer near its resonant frequency f 0 and kept at a constant height Δ h above the surface. When the tip is placed in proximity to a sample, the cantilever’s resonant motion is altered in ways that can be traced directly to the force gradient ∂ F z /∂ z , which in turn produces changes in the amplitude Δ A , phase Δ φ and frequency Δ f of the cantilever resonance [26] , [29] : In equation (1, 2, 3), k is the spring constant of the cantilever and Q ≈136 is the quality factor of the resonance. Force gradients may arise from magnetic or non-magnetic interactions, so it is important to conduct experiments that can distinguish the two sources of contrast. MFM images on top electrode MFM imaging using frequency modulation [29] is performed directly over the top electrode ( Fig. 1a ). The MFM tip and top gate are both grounded, eliminating any possible electrostatic coupling. The topographic image in Fig. 1b has nanometer-scale surface roughness associated with inhomogeneity in the Au layer. The tip is magnetized perpendicular to the LAO/STO interface and cantilever frequency-shift images are obtained for conducting ( V dc =0 V, Fig. 1c ) and insulating ( V dc =−2 V, Fig. 1d ) states of the LAO/STO interface. The frequency shift is negligibly small for both voltage gating conditions, with the exception of a few topographic features. The root mean square frequency shift is Δ f =0.43 Hz for V dc =0 V and Δ f =0.44 Hz for V dc =−2 V, close to the noise floor of 0.27 Hz for the measurement. The tip is then magnetized along the in-plane [010] orientation, and frequency-shift images are acquired with the same tip, over the same region on the sample, under the same voltage bias conditions as with Fig. 1c,d . In the conductive state ( V dc =0 V, Fig. 1e ), the image shows negligible spatial variations in the frequency shift. In the insulating state ( V dc =−2 V, Fig. 1f ), the frequency-shift image shows significant contrast, of the order 20 Hz peak-to-peak (note the change in frequency-shift scale). The calculated force gradient magnitude, based on equation (3) and the cantilever properties ( Supplementary Fig. 4 ), is of the order 10 −4 N m −1 . The boundaries between domains of approximately equal frequency shift are sharp, straight and aligned ~30–40° relative to the horizontal axis. Experiments performed at various angles between the MFM tip and the sample show that the stripe contrast is maximized for tip magnetization oriented along the [100] or [010] direction, and vanishes for tip magnetizations that approach the [110] and directions ( Supplementary Fig. 8 , Supplementary Note 2 ). Experiments performed with a non-magnetic tip show no visible contrast at any gate voltage in the range −3–+3 V ( Fig. 2 ). 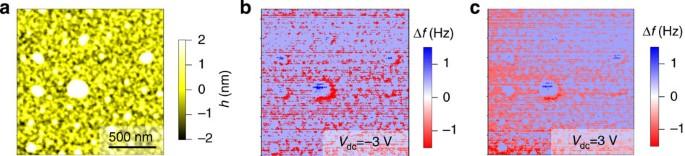Figure 2: Control MFM experiments using non-magnetic tip on top electrode over a 1.5 × 1.5 μm area. (a) Height image. (b) MFM frequency image withVdc=−3 V andVdc=3 V. Results are shown for Device A. Tip is driven at its resonant frequencyω0/2π=70 kHz at a height Δh=20 nm above the top electrode surface. Figure 2: Control MFM experiments using non-magnetic tip on top electrode over a 1.5 × 1.5 μm area. ( a ) Height image. ( b ) MFM frequency image with V dc =−3 V and V dc =3 V. Results are shown for Device A. Tip is driven at its resonant frequency ω 0 /2 π =70 kHz at a height Δ h =20 nm above the top electrode surface. Full size image The experiments described above provide compelling evidence for a ferromagnetic phase localized at the LAO/STO interface. The MFM tip is electrically screened by the grounded top electrode, thus ruling out contrast mechanisms that are electrical in nature. Furthermore, the strong sensitivity of the MFM contrasts to the magnetization direction of the tip, holding all other experimental parameters fixed, providing compelling evidence for a magnetic interaction with an in-plane magnetized phase. MFM images over LAO close to top electrode The experiments described so far are performed over the Ti/Au-coated LAO/STO heterostructure. To help understand possible contributions associated with the metal deposition itself, as well as possible local leakage currents from the top electrode, MFM experiments are also performed directly over the LAO surface in a region ~10 μm from the edge of the circular top electrode ( Fig. 3a ). The exposed LAO surface is atomically flat with clearly-resolved single-unit-cell 0.4 nm steps. To check that electrical gating is possible several micrometers away from the circular electrode edge, the surface potential is mapped using Kelvin-probe force microscopy. 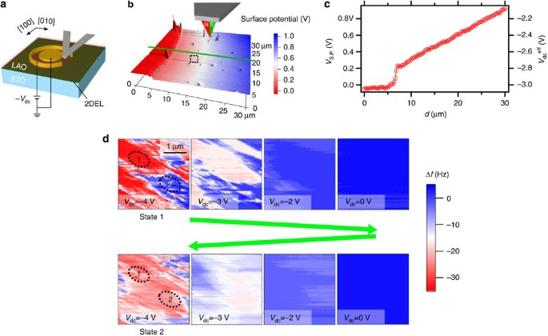Figure 3: MFM experiments performed over the exposed LAO region. (a) experimental set-up, similar to that ofFig. 1a, except the scanning location is now over the exposed LAO surface, ~10 μm away from the electrode edge. (b) Kelvin-probe force microscopy measurement of a region that includes the area for which MFM measurements are made. The top gate is grounded and voltage bias to the interface (−Vdc) is 3 V. The topography is shown as height, while the colour maps onto the measured surface potential (the work function is already subtracted). (c) Surface potential profile along the green linecut inb. showing that the voltage gating decays but is reduced by ~1 V in the area over which MFM images are acquired. HereVdceffis defined as the potential difference between surface and interface:Vdceff=Vs.p.−(−Vdc)=Vs.p.+Vdc. (d) MFM frequency images over a 3 × 3 μm area indicated by the black dashed line enclosed region inb. The MFM tip is magnetized horizontally parallel to the [010] sample direction. MFM frequency images forVdcincreasing from −4 to 0 V then decreasing to −4 V. Magnetic domain features are clearly observed forVdc<−2 V. The final State 2, obtained after cycling the voltage toVdc=0, is uncorrelated from the initial State 1. The regions enclosed by dashed lines give example of where magnetic contrast is unchanged (region 1) or reversed (region 2) after voltage cycling. Figure 3b shows the surface potential distribution over the investigated area with the top gate grounded and the interface biased at 3 V. (The work function difference between the metal top gate and the LAO surface is accounted for, and described in Supplementary Fig. 9 ). A cross-sectional profile analysis shows that the electrode-induced top gating decays gradually over tens of micrometers from the top electrode edge ( Fig. 3c ). Within the rectangular area marked by a dashed line, MFM measurements are performed as a function of gate voltage ( Fig. 3d ). The first MFM image, taken at V dc =−4 V (‘State 1’), shows strong contrast in the frequency channel similar to that seen over the electrode. No correlation of the frequency shift with unit-cell terraces is observed. As the gate bias is increased, the contrast between domains diminishes. For V dc =−2 V, the domain contrast has nearly vanished with new horizontal bands appearing parallel to the fast scan axis. For V dc =0, the contrast is absent. Subsequent decrease of V dc restores the magnitude of the response but with a new domain pattern that is uncorrelated with the previous one (‘State 2’). The observed magnetic contrast away from the electrode is qualitatively consistent with images taken directly over top electrode, indicating that neither surface leakage currents nor metal/oxide chemistry is responsible for the magnetism. (Similar results are also shown for Device B and C in Supplementary Fig. 10 ). The slight decrease in magnitude is correlated with charge hysteresis in the CV spectrum ( Supplementary Fig. 2 ) during voltage gate sweeps. Figure 3: MFM experiments performed over the exposed LAO region. ( a ) experimental set-up, similar to that of Fig. 1a , except the scanning location is now over the exposed LAO surface, ~10 μm away from the electrode edge. ( b ) Kelvin-probe force microscopy measurement of a region that includes the area for which MFM measurements are made. The top gate is grounded and voltage bias to the interface (− V dc ) is 3 V. The topography is shown as height, while the colour maps onto the measured surface potential (the work function is already subtracted). ( c ) Surface potential profile along the green linecut in b . showing that the voltage gating decays but is reduced by ~1 V in the area over which MFM images are acquired. Here V dc eff is defined as the potential difference between surface and interface: V dc eff = V s.p. −(− V dc )= V s.p. + V dc . ( d ) MFM frequency images over a 3 × 3 μm area indicated by the black dashed line enclosed region in b . The MFM tip is magnetized horizontally parallel to the [010] sample direction. MFM frequency images for V dc increasing from −4 to 0 V then decreasing to −4 V. Magnetic domain features are clearly observed for V dc <−2 V. The final State 2, obtained after cycling the voltage to V dc =0, is uncorrelated from the initial State 1. The regions enclosed by dashed lines give example of where magnetic contrast is unchanged (region 1) or reversed (region 2) after voltage cycling. Full size image Magnetization re-orientation in successive MFM scan The observed large-scale domain structures in the MFM images are generally reproducible from one scan to the next ( Fig. 4a,b ), but there are differences in fine domain structures from successive scans that suggest tip-induced magnetization switching. The subtle changes from images acquired in succession are readily seen by examining the phase error channel Δ φ ( Fig. 4c,d ), which is used to maintain a constant phase shift between the driving signal and the tip response. Acting as a high-pass spatial filter, the phase error image accentuates sharp features in the MFM images. A line cut perpendicular to the domain boundaries ( Fig. 4e ) shows that the first image taken at V dc =−2 V exhibits domains that are as narrow as 30 nm in width; this fine domain structure is largely absent in the subsequently acquired image. Considering the fact that the MFM experiments are operated in non-contact mode and the tip never comes in contact with the surface, the observed magnetic re-orientation of the sample is most likely due to magnetization re-orientation from the magnetic tip. 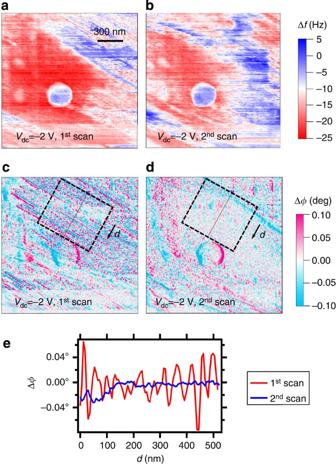Figure 4: MFM images acquired in succession. (a,b) two successive MFM frequency images and corresponding phase offset images withVdc=−2 V. (c,d) the corresponding phase error images. (e) Averaged line scans (in the dashed box) perpendicular to domain patterns for two successive scans atVdc=−2 V illustrate how the fine domain structure is altered by the MFM tip. Stripe domains with widths as small as 30 nm, observed in the first scan, are no longer present in the subsequent scan. Figure 4: MFM images acquired in succession. ( a , b ) two successive MFM frequency images and corresponding phase offset images with V dc =−2 V. ( c , d ) the corresponding phase error images. ( e ) Averaged line scans (in the dashed box) perpendicular to domain patterns for two successive scans at V dc =−2 V illustrate how the fine domain structure is altered by the MFM tip. Stripe domains with widths as small as 30 nm, observed in the first scan, are no longer present in the subsequent scan. Full size image Dynamic magneto-electric force microscopy (MeFM) mapping The gate dependence of the MFM images demonstrates a strong interaction between ferromagnetism and itinerant electrons. To help explore this connection, we perform dynamic MeFM experiments ( Fig. 5a ). With MeFM, the tip is not mechanically driven; instead, the interface potential is electrically modulated at the mechanical resonance of the cantilever, and the resulting AC magnetic field from the LAO induces resonant motion of the magnetized cantilever. The surface topography image is included in Fig. 5b . MeFM amplitude images ( Fig. 5c ) are acquired at values of V dc ranging between −3.5 and 0 V. As the carrier density increases, the contrast in MeFM images becomes weaker and more diffuse. Similar contrast is also observed in MeFM images taken over the top electrode ( Supplementary Figs 11–12 ) and more MeFM images over LAO near the top gate ( Supplementary Figs 13–14 , Supplementary Note 3 ). The observed stripe domains and the contrast changes in MeFM images agree qualitatively with the results obtained by conventional MFM imaging. The coupling of the magnetic response to carrier density establishes that the electrons entering the interface become spin-polarized, aligning antiferromagnetically with the magnetic domains. Additional scan sequences ( Supplementary Figs 13–14 ) show that voltage hysteresis in the magnetic response can be traced back to observed hysteresis in the CV spectrum ( Supplementary Fig. 2 ). 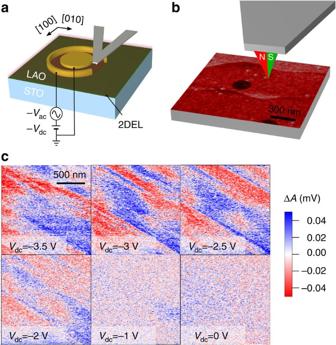Figure 5: Magneto-electric force microscopy experiments above the exposed LAO surface near the top electrode. (a) Sketch of the experimental set-up. A combined AC and DC bias is applied to the interface with the top gate grounded. The AC bias is at a fixed frequency equal to the cantilever’s free resonant frequency. Unlike MFM, the tip is not driven mechanically. The tip is electrically isolated and kept at a constant height above the sample surface during imaging. (b) Topographic image of the sample where magneto-electric force microscopy (MeFM) images are acquired. Image size is 1.5 × 1.5 μm about ~5 μm away from the edge of the top electrode. (c) MeFM amplitude images acquired withVdcincreasing from −3.5 to 0 V. Each image is shown with the average value subtracted: 0.26 mV, 0.19 mV, 0.14 mV, 0.09 mV, 0.06 mV, 0.07 mV, respectively. Figure 5: Magneto-electric force microscopy experiments above the exposed LAO surface near the top electrode. ( a ) Sketch of the experimental set-up. A combined AC and DC bias is applied to the interface with the top gate grounded. The AC bias is at a fixed frequency equal to the cantilever’s free resonant frequency. Unlike MFM, the tip is not driven mechanically. The tip is electrically isolated and kept at a constant height above the sample surface during imaging. ( b ) Topographic image of the sample where magneto-electric force microscopy (MeFM) images are acquired. Image size is 1.5 × 1.5 μm about ~5 μm away from the edge of the top electrode. ( c ) MeFM amplitude images acquired with V dc increasing from −3.5 to 0 V. Each image is shown with the average value subtracted: 0.26 mV, 0.19 mV, 0.14 mV, 0.09 mV, 0.06 mV, 0.07 mV, respectively. Full size image The MFM tip strongly perturbs the magnetic domain structure, as can be seen from successive scans (for example, Fig. 4 ). Angle-dependent MFM measurements ( Supplementary Fig. 8 ) can be interpreted as evidence for in-plane anisotropy along the [100] and [010] directions, but it is more likely that the domains are aligned along the [110] and directions, with domain structure that is stable against perturbation from the MFM tip only close to θ =0°. The domain walls themselves are generally sharp and resolution limited, with apparent widths that depend on V dc ( Supplementary Fig. 15 , Supplementary Note 4 ). The absence of features in MFM images with vertically magnetized tips ( Fig. 1c,d ) have several possible explanations. One is that the domain walls are Néel-type, with magnetization rotating in the plane of the sample or vanishing at the domain wall [30] . An alternate explanation is that the magnetization of the tip is too strongly perturbing the domain state to allow them to be imaged. A third possibility is that the domain walls are too narrow to be detected. Theories of magnetism at the LAO/STO interface generally invoke localized unpaired d xy electron spins at the interface that couple via exchange with itinerant carriers. The mechanism depends on the relative density of localized versus itinerant electrons, as well as their orbital character [20] , [31] , [32] . Fidkowski et al . [32] describe a ferromagnetic Kondo model in which local d xy moments couple ferromagnetically to delocalized d xz / d yz carriers; models with ferromagnetic exchange are also described by Joshua et al . [20] and Bannerjee et al . [33] Michaeli et al . [34] describe a model based on Zener (antiferromagnetic) exchange between localized and delocalized d xy carriers [35] . The local moments themselves are postulated to arise either from electronic correlations [36] or interfacial disorders [32] , [34] , or are related to oxygen vacancies [31] , [37] . Extrinsic sources of magnetic impurities have been ruled out experimentally [11] , [12] , [15] . From the histogram analysis of MFM images across the magnetic domain boundary ( Supplementary Fig. 16a–b ), the net magnetization is greatly reduced as the carrier density increases ( Supplementary Fig. 16c ). The averaged frequency signal of the MFM images with varied V dc ( Supplementary Fig. 17 ) shows a rapid drop as V dc decreases ( Supplementary Fig. 17d and Supplementary Note 5 ), which suggests that the net magnetization increases as the carrier density depletes. These analyses indicate that the exchange is primarily antiferromagnetic and distinct from the Kondo-related [38] ferromagnetism [39] reported for electrolyte-gated STO. The source of the local moments is not obviously constrained by these experiments, except for the fact that they appear to be highly uniform-domain walls that are sharp and highly linear and not pinned by fluctuations in moment density. The two growth conditions explored here (see Table S1 ) are both believed to have a low density of oxygen vacancies near the interface. The existence of room-temperature ferromagnetism at the insulating LAO/STO interface offers a pathway to resolve many of the contradictory reports regarding magnetism at the LAO/STO interface. Most experimental investigations have been performed with conducting interfaces, a regime for which higher-temperature ferromagnetism is suppressed. Any inhomogeneity that locally depletes the interface, for example, defects or surface adsorbates [24] , could give rise to local insulating regions that exhibit magnetic behaviour. Similarly, LAO/STO structures grown at pressures close to the insulating transition (for example, P(O 2 )=10 −2 mbar for ref. 12 ) may contain local insulating regions that exhibit room-temperature ferromagnetic behaviour. Experiments by Kalisky et al . [40] suggest that there could be a critical LAO thickness below which magnetism is not observed. At higher carrier densities (and lower temperatures), a distinct class of magnetic behaviour is observed, with signatures such as anomalous Hall effect, anisotropic magnetoresistance and coexistence of superconductivity. Above the Lifshitz transition, local moments are predicted to align ferromagnetically with the d xz / d yz electrons, from Hund’s rule coupling [20] , [32] , [33] . Such properties are distinct from the room-temperature ferromagnetism reported here. There are many unresolved questions regarding the nature of the ferromagnetic state. First and foremost, the density of localized moments, and the relative density of delocalized carriers, is not well-characterized by these MFM measurements. The magnetic moment density is a quantity that in principle can be obtained from MFM measurements but is challenging here given the fact that the magnetization is so strongly perturbed by the MFM tip. The magnetic easy axes are not readily identified, although there is clear in-plane magnetic anisotropy. Future refinements of these experiments as well as new ones will undoubtedly answer these questions and help to constrain theoretical descriptions. To sum up, we use both MFM and MeFM to search the magnetism on gated LAO/STO systems at room temperature. An in-plane ferromagnetic phase emerges as electrons are depleted from the interface and vanishes as the interface is modulated to be conducting. Controlled experiments with non-magnetic probe ( Fig. 2 and Supplementary Fig. 18 ) indicates that the observed MFM signal contrast is magnetic in nature and MFM experiments on pure STO ( Supplementary Fig. 19 ) shows no magnetic defects in the STO substrate. The discovery of electrically controlled ferromagnetism at the LAO/STO interface at room temperature provides a new and surprising route to a wide range of spintronics applications. Many effects—not yet demonstrated—are nevertheless expected, such as spin-torque transfer, spin-polarized transport, electrically controlled spin-wave propagation and detection, magnetoresistance effects and spin-transistor behaviour. This versatile spintronic functionality may also be combined with conductive AFM control over the metal-insulator transition [25] , both for room-temperature spintronics applications and low-temperature quantum devices. Sample growth and device fabrication Samples are grown by pulsed laser deposition. Before deposition, low-miscut (<0.1°) STO substrates are etched using buffered hydrofluoric acid to keep the TiO 2 -termination. Then the STO substrates are annealed at 1,000 °C for several hours so the atomically flat surfaces are created. During the deposition, a KrF exciter laser ( λ =248 nm) beam is focused on a stoichiometric LAO single crystal target with energy density 1.5 J cm −2 and each LAO unit cell is deposited by 50 laser pulses. Two different growth conditions are used for the substrate growth temperate T and chamber background partial oxygen pressure P (O 2 ): (1) T =550 °C and P (O 2 )=10 −3 mbar; (2) T =780 °C, P (O 2 )=10 −5 mbar. For samples grown in condition (2), after deposition they are annealed at 600 °C in P (O 2 )=300 mbar for 1 h to minimize oxygen vacancies. Device fabrication The fabricated device is a two-terminal capacitor structure, consisting of a circular top electrode and an electrode contacting the LAO/STO interface. As shown in Fig. 1a , the electrodes contacting the interface are arc-shaped with a width of 20 μm and fixed separation of 50 μm to the edge of the circular top gates. The capacitor electrodes are deposited on the LAO/STO samples via direct current sputtering. The arc-shaped electrodes are prepared by creating 25 nm trenches via Ar-ion milling, followed by deposition of 4 nm of Ti and 30 nm of Au. A series of metallic circular top gates (4 nm Ti and 40 nm Au) are deposited on the LAO surface. The entire sample (5 × 5 × 0.5 mm) is affixed to a ceramic chip carrier using silver paint. Electrical contacts to bonding pads on the device are made with an ultrasonic wire bonder using gold wires. The investigated devices with parameters are summarized in Supplementary Table 1 . Magnetic force microscopy The CoCr-coated tip is magnetized with electromagnets. The cantilever has a resonant frequency f 0 ≈70 kHz; in MFM mode, the tip first measures the topographic profile and then scans at a constant height Δ h above the surface to get the MFM signal. Conventional dynamic MFM is performed using either frequency modulation [29] or slope detection [26] . In the main text, frequency modulation method is employed. A 90° phase shift between cantilever drive and response is maintained using a feedback loop. During scanning, the tip is raised at a constant height Δ h above the surface to reduce the effects of topography on MFM signal. In Figs 1 , 4 , the tip height over the top electrode is 30 nm and the scan area on top electrode is a 1.4 μm square. For the MFM experiments above the exposed LAO surface ( Fig. 3 ), the tip-surface separation is Δ h =20 nm and the scan size is 3 μm. In Figs 1 , 2 , 3 , 4 , the cantilever’s drive frequency is ω 0 /2 π =70 kHz. The amplitude, phase and frequency shift are all recorded for various values of V dc . Magneto-electric force microscopy The MeFM technique was used to image the coupling between the magnetic and electric dipoles in magneto-electric materials [41] . Here MeFM method is employed to explore the connection between ferromagnetism and itinerant electrons. Rather than driving the tip mechanically, the sample is driven with a static and sinusoidally modulated voltage. The gate-modulated sample magnetization periodically changes the magnetic force, driving the tip resonantly and producing a cantilever oscillation that is detected with a lock-in amplifier. Figure 5 in the main text shows the MeFM experiments with the tip scanned above the LAO close to the top electrode. The tip remains magnetized along the [010] direction. The top electrode is grounded to minimize electrostatic interactions between the tip and the sample, and a combined voltage is applied to the interface V IF ( t )=−( V dc + V ac sin(2π ft )), with V ac =0.14 V and f =70.6 kHz. The tip is maintained at a distance of 20 nm above the LAO surface and scanned over a 1.5 μm square area on Device A. The deflection signal from the tip is monitored by a lock-in amplifier at the resonant frequency f . How to cite this article: Bi, F. et al . Room-temperature electronically-controlled ferromagnetism at the LaAlO 3 /SrTiO 3 interface. Nat. Commun. 5:5019 doi: 10.1038/ncomms6019 (2014).